Transparency and damage tolerance of patternable omniphobic lubricated surfaces based on inverse colloidal monolayers A transparent coating that repels a wide variety of liquids, prevents staining, is capable of self-repair and is robust towards mechanical damage can have a broad technological impact, from solar cell coatings to self-cleaning optical devices. Here we employ colloidal templating to design transparent, nanoporous surface structures. A lubricant can be firmly locked into the structures and, owing to its fluidic nature, forms a defect-free, self-healing interface that eliminates the pinning of a second liquid applied to its surface, leading to efficient liquid repellency, prevention of adsorption of liquid-borne contaminants, and reduction of ice adhesion strength. We further show how this method can be applied to locally pattern the repellent character of the substrate, thus opening opportunities to spatially confine any simple or complex fluids. The coating is highly defect-tolerant due to its interconnected, honeycomb wall structure, and repellency prevails after the application of strong shear forces and mechanical damage. The regularity of the coating allows us to understand and predict the stability or failure of repellency as a function of lubricant layer thickness and defect distribution based on a simple geometric model. Motivated by a broad potential impact on science and technology, the design of liquid-repellent surfaces has been the subject of intense research that has led to the development of superhydrophobic [1] , [2] , [3] , [4] and, more recently, superomniphobic [5] , [6] , [7] , [8] , [9] surface coatings, which show resistance to water and organic liquids, respectively. The design of such surfaces has been adapted from nature’s famously self-cleaning lotus leaves [10] . The underlying design principle is the reduction of contact points of a liquid droplet by the introduction of roughness features. Thus, a solid/air composite surface is created [11] that enables liquid droplets to roll off with ease. Despite remarkable improvements in liquid repellency [5] , [6] , [7] , [8] , transparency [7] , [12] and durability [7] , [13] made possible by increasingly sophisticated surface microstructure designs, several challenges remain: most importantly, the adsorption of proteins or bacteria to superhydrophobic surfaces [14] , [15] , pressure instability [16] , [17] , limited self-healing properties and the impossibility of creating thermodynamically stable non-wetting states for low-surface-tension liquids [6] . The development of lubricant-infused porous materials, inspired by nature’s Nepenthes pitcher plant [18] , has recently introduced a new paradigm for the creation of surfaces with the capability to repel arbitrary aqueous and organic liquids [19] . In contrast to the lotus-inspired approach, these slippery liquid-infused porous surfaces (SLIPS) are designed to create a fluid/fluid interface between a lubricant and the immiscible liquid to be repelled. To maintain stable repellency, such a surface needs to be optimized in a way that the lubricant layer is not displaced from the solid’s surface: if the free energy of the solid/lubricant/liquid system is minimal for the situation where the test liquid resides on the lubricant layer without replacing it, the liquid/liquid interface effectively eliminates pinning points, leading to super-repellent surfaces with extremely low sliding angles—even for liquids with very low surface tensions. Additionally, the fluid nature of the interface possesses self-healing characteristics, allows for remarkable pressure-stability [19] and has been shown to effectively prevent the attachment of bacteria [20] and ice [21] , thus overcoming many of the challenges of conventional repellent surfaces. Though conceptually different, both lotus-inspired and SLIPS designs require roughness to support repellency. For a SLIPS surface, this roughness—paired with surface functionalization to match the chemical nature of the lubricant—allows effective confinement of the lubricant inside the structured solid. In initial attempts, perfluorinated lubricants were wicked into porous Teflon membranes that provided both matching fluorinated surface functionalities as well as a nanoporous confinement. [19] Additionally, chemically functionalized micron-scale roughness features prepared by conventional and soft lithography [19] , [20] , [22] , [23] , electrodeposition of polypyrrole nanostructures [21] and sol-gel derived aluminium oxide nanostructures [24] , [25] have recently been successfully employed as structured solids for lubricant infiltration. Here we report on the design of a fully transparent SLIPS coating based on colloidal templating [26] , [27] , [28] , [29] . In our approach, a colloidal monolayer is backfilled by a silica precursor to form an inverse replica that serves as a porous layer to lock-in the lubricant. There are multiple reasons to employ colloids as building blocks. The regular arrangement of colloids in a monolayer [30] is experimentally simple, fast and cheap and gives access to nanopores of well-defined size, shape and order, thus allowing us to precisely calculate and control surface roughness. In contrast to irregular nanostructures, this enables a fundamental analysis of the stability of a liquid-infused coating based on geometric models. The silica backfilling allows for strong, covalent bonding of the nanostructured film to glass or oxide substrates, preventing delamination or adhesive failure of the film and thus enhancing the robustness of the surface structures. Additionally, it can be modified by well-developed silane chemistry that provides a broad range of stable, covalently bound monolayers terminated with surface functionalities matched to the properties of the lubricant. The tunability of pore sizes at the nanometre scale can be used to engineer the optical properties of materials across a wide range of wavelengths and enables the formation of transparent surface coatings [12] , a prerequisite, for example, for the application of SLIPS to windows or solar cells. Homogeneity and chemical resistance of the colloid-templated silica coating allows for the application of conventional photolithography to pattern the repellent character of the surface. The combination of the strong liquid repellency of a SLIPS coating with surface patterning protocols is of high practical interest as it may open pathways to confine low-surface-tension liquids (for example, oil) and complex fluids (for example, blood) to designated parts of a surface. This novel methodology could be implemented to create SLIPS-based microfluidic devices that operate without solid interfaces or could be used to confine small blood droplets into microscopic arrays, for example, for medical diagnostics [31] , [32] . Surface structure design and liquid repellency The key challenge in designing highly repellent lubricant-infused structured surfaces by colloidal templating is the ability to homogeneously cover large areas of solid substrates with colloidal monolayers. In our approach, we preassemble colloids at the air/water interface and subsequently transfer them to the desired substrates [33] , [34] . The liquid nature of the interface provides fluidity necessary to achieve high order and uniform coverage and inherently confines the colloids to a two-dimensional layer. This avoids the formation of multilayers that might act as pinning points for applied test liquids and compromise repellency. Additionally, the process allows for uniformly depositing colloidal monolayers over large areas, limited only by the dimensions of the water’s surface, and is able to cover curved or topographically structured surfaces [33] , [34] , [35] . 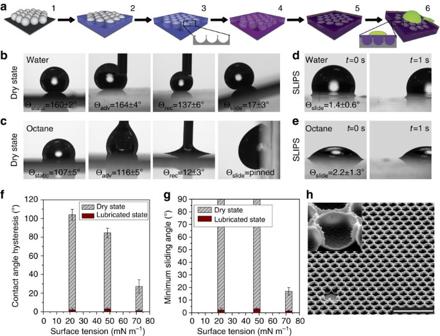Figure 1: Lubricant-infused inverse monolayers as omniphobic super-repellent surfaces. (a) Construction scheme: after assembly on the desired surface (1), the colloidal monolayer is backfilled with silica precursor solution of tetraethylorthosilicate (TEOS) (2), and the organic colloids are combusted to give rise to an inverse structure composed of silica (3). Fluorosilanization of the surface with, for example, (1H,1H,2H,2H-tridecafluorooctyl)-trichlorosilane (4) matches the surface chemistry of the inverse colloidal structure to the chemical nature of the perfluorinated lubricant (DuPont Krytox 100) that consequently wicks into the porous network and forms a stable liquid film held in place by the nanostructures (5). A liquid droplet immiscible with the fluorocarbon lubricant will be effectively repelled (6). (b,c) Wetting of dry, fluorosilanized substrates with water (b) and octane (c). From left to right, the images show static and dynamic (advancing and receding) contact angles as well as the minimum tilt angle required for the droplet movement. The dry substrate shows superhydrophobic behavior with high dynamic contact angles and low roll-off angles of a water droplet. An octane droplet is strongly pinned to the substrate and thus features an extremely low receding contact angle. As a consequence, it cannot slide off the substrate even if placed vertically, indicating the failure of the dry substrate to repel octane. (d,e) Wetting properties after infiltration with fluorinated lubricant: time-lapsed images show very low sliding angles of water (d) and octane (e) resulting from the absence of pinning points at the lubricant/liquid interface and thus demonstrate efficient repellency of both liquids. (f,g) Quantification of the omniphobic behavior with liquids of decreasing surface tensions (water, ethylene glycol and octane). The SLIPS state is characterized by extremely low contact angle hysteresis (f) and sliding angles (g) for all tested liquids, while dry samples induce pinning of all liquid droplets except water. All values were averaged over 10 individual measurements. The error bars represent the standard deviation of 10 individual measurements. (h) SEM image taken at an angle of 45° showing high regularity and structural details of the nanopore arrays. The scale bar is 5 μm. Figure 1a schematically shows the construction of a SLIPS coating from a colloidal template. Structural details and the high uniformity and regularity of the prepared nanoporous layer can be seen in SEM images ( Fig. 1h and Supplementary Fig. S1 ). Figure 1b–g compares the wetting properties of the nanostructured surfaces made from 1 μm colloids in dry and lubricated states. The dry, fluorinated structures show superhydrophobic characteristics [27] with high dynamic contact angles and reasonably low sliding angles ( Fig. 1b ). However, they fail to repel low-surface-tension octane: a withdrawing droplet is strongly pinned to the surface, leading to an extremely high contact angle hysteresis, and will not slide off the substrate even when placed vertically ( Fig. 1c ). When the same substrate is infused with a fluorinated lubricant, drastic changes are observed: the complete elimination of pinning points induces super-repellency with high droplet mobility that leads to extremely low sliding angles for both water and octane ( Fig. 1d,e ). A quantitative assessment of contact angle hysteresis and minimum sliding angles (5 μl droplet) for liquids with a range of surface tensions (water, ethylene glycol and octane) shown in Fig. 1f,g further highlights the significant differences between the dry and lubricated states and reveals the highly efficient repellency of the SLIPS coating compared to its superhydrophobic analogue. It is noteworthy that the repellent properties of these surfaces are not limited to the use of fluorinated liquids as lubricants: with a proper adjustment of the surface chemistry, a variety of different fluids can be used as lubricants to repel a second, immiscible liquid. As examples, we show the water-repellent properties of hexadecane- and olive oil-infused coatings functionalized with hydrophobic decyltrichlorosilane molecules or, more remarkably, the repellency of the fluorinated oil itself by water-infused hydrophilic inverse monolayers ( Supplementary Fig. S2 , Supplementary Movie 1 ). Figure 1: Lubricant-infused inverse monolayers as omniphobic super-repellent surfaces. ( a ) Construction scheme: after assembly on the desired surface (1), the colloidal monolayer is backfilled with silica precursor solution of tetraethylorthosilicate (TEOS) (2), and the organic colloids are combusted to give rise to an inverse structure composed of silica (3). Fluorosilanization of the surface with, for example, (1H,1H,2H,2H-tridecafluorooctyl)-trichlorosilane (4) matches the surface chemistry of the inverse colloidal structure to the chemical nature of the perfluorinated lubricant (DuPont Krytox 100) that consequently wicks into the porous network and forms a stable liquid film held in place by the nanostructures (5). A liquid droplet immiscible with the fluorocarbon lubricant will be effectively repelled (6). ( b , c ) Wetting of dry, fluorosilanized substrates with water ( b ) and octane ( c ). From left to right, the images show static and dynamic (advancing and receding) contact angles as well as the minimum tilt angle required for the droplet movement. The dry substrate shows superhydrophobic behavior with high dynamic contact angles and low roll-off angles of a water droplet. An octane droplet is strongly pinned to the substrate and thus features an extremely low receding contact angle. As a consequence, it cannot slide off the substrate even if placed vertically, indicating the failure of the dry substrate to repel octane. ( d , e ) Wetting properties after infiltration with fluorinated lubricant: time-lapsed images show very low sliding angles of water ( d ) and octane ( e ) resulting from the absence of pinning points at the lubricant/liquid interface and thus demonstrate efficient repellency of both liquids. ( f , g ) Quantification of the omniphobic behavior with liquids of decreasing surface tensions (water, ethylene glycol and octane). The SLIPS state is characterized by extremely low contact angle hysteresis ( f ) and sliding angles ( g ) for all tested liquids, while dry samples induce pinning of all liquid droplets except water. All values were averaged over 10 individual measurements. The error bars represent the standard deviation of 10 individual measurements. ( h ) SEM image taken at an angle of 45° showing high regularity and structural details of the nanopore arrays. The scale bar is 5 μm. Full size image Optical properties The pore size of the inverse monolayers was adjusted from 140 to 1,060 nm by changing the colloid size while maintaining close-packed order and regularity ( Fig. 2a ). Downscaling the structure sizes has strong effects on the optical properties. 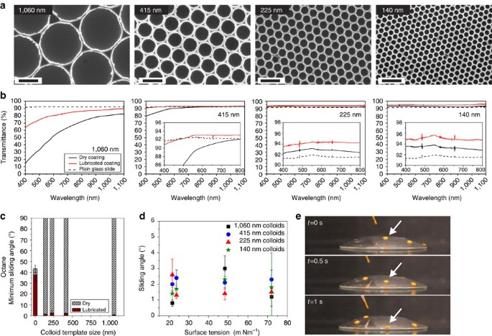Figure 2: Optical properties and liquid repellency for substrates with different colloid template sizes. (a) SEM images showing the ability to create inverse monolayer structures down to a size of 140 nm (the colloid sizes are indicated in the top left corner). All scale bars are 500 nm. (b) Optical properties of microscope slides covered with inverse monolayers in dry (black lines) and lubricated (red lines) state. Full transparency is achieved with feature sizes of <415 nm. Inverse monolayer structures with feature sizes of 225 nm and 140 nm show enhanced transmittance of light over the full visible spectrum (see insets). (c,d) Wetting properties, characterized by the minimum angle required to remove a liquid droplet (sliding angle) of the differently sized inverse monolayers in dry and lubricated states for octane as a probe liquid (left side) and for water, ethylene glycol and octane in the lubricated state (right side). SLIPS conditions are maintained for all structure sizes and all liquids tested. All values were averaged over 10 individual measurements. The error bars represent the standard deviation of 10 individual measurements. (e) Super-repellent properties of a SLIPS coating applied to a curved substrate, shown for a watch glass (d=10 cm) as an example (seeSupplementary Movie 2). The SLIPS character is demonstrated by time-lapsed images showing the effective repellency of dyed octane droplets (highlighted by white arrows). Figure 2b compares UV-Vis-NIR transmission spectra of the differently sized inverse monolayers deposited on one side of microscope slides at normal incidence in dry (black lines) and lubricated states (red lines), and to untreated glass slides (dotted black lines). The large colloids (1,060 nm) show a strong coloration arising from Mie resonances of the individual structures and diffractively coupled resonances of the ordered structures [36] . With decreasing feature size, light losses are strongly diminished and the substrate’s transparency is identical to a plain glass slide used as a control. The addition of the lubricant decreases the refractive index contrast, leading to a drastic reduction in light losses. From a colloid template size of 415 nm, no loss of transmitted light intensity is detected and the substrates appear as transparent as regular glass slides. For colloid template sizes of 225 nm and 138 nm, the SLIPS coating leads to enhanced light transmission of up to 3%. We attribute the enhanced transmission to the reduced refractive index contrast of the lubricant/air interface compared to the original glass/air interface. Figure 2: Optical properties and liquid repellency for substrates with different colloid template sizes. ( a ) SEM images showing the ability to create inverse monolayer structures down to a size of 140 nm (the colloid sizes are indicated in the top left corner). All scale bars are 500 nm. ( b ) Optical properties of microscope slides covered with inverse monolayers in dry (black lines) and lubricated (red lines) state. Full transparency is achieved with feature sizes of <415 nm. Inverse monolayer structures with feature sizes of 225 nm and 140 nm show enhanced transmittance of light over the full visible spectrum (see insets). ( c , d ) Wetting properties, characterized by the minimum angle required to remove a liquid droplet (sliding angle) of the differently sized inverse monolayers in dry and lubricated states for octane as a probe liquid (left side) and for water, ethylene glycol and octane in the lubricated state (right side). SLIPS conditions are maintained for all structure sizes and all liquids tested. All values were averaged over 10 individual measurements. The error bars represent the standard deviation of 10 individual measurements. ( e ) Super-repellent properties of a SLIPS coating applied to a curved substrate, shown for a watch glass ( d =10 cm) as an example (see Supplementary Movie 2 ). The SLIPS character is demonstrated by time-lapsed images showing the effective repellency of dyed octane droplets (highlighted by white arrows). Full size image The influence of the feature size of the surface structure on the liquid repellency was assessed by measurements of the minimum sliding angle of octane in dry and lubricated states ( Fig. 2c ) and the corresponding contact angle hysteresis ( Supplementary Fig. S3 ). A strong difference in wetting characteristics can be seen for all colloid template sizes. Dry samples show pinning of the droplet and high contact angle hysteresis. After lubrication all structure sizes support high repellency, with contact angle hysteresis and sliding angles not exceeding 5°. The SLIPS state is maintained for all colloid template sizes with all liquids tested ( Fig. 2d ). It is noteworthy that although the size of the pores does not affect the SLIPS characteristics, reference measurements performed on lubricated, fluorinated, flat samples without surface nanostructures show higher contact angle hysteresis and sliding angles, thus suggesting that the presence of the underlying surface roughness is required for efficient repellency. We further demonstrate that transparent slippery coatings based on inverse colloidal monolayers can be easily applied to curved substrates, thus providing a self-cleaning coating for optical windows. Figure 2e shows time-lapsed images (taken from Supplementary Movie 2 ) of a watch glass covered with an inverse monolayer-based SLIPS coating that repels dyed octane droplets. Likewise, the curved surface of a glass vial was rendered slippery and showed perfect non-wetting behavior when immersed in dyed octane or water solutions ( Supplementary Fig. S4 and Supplementary Movie 3 ). Adhesion prevention In general, a major source of surface contamination arises from adsorption of liquid-borne contaminants to a solid surface in contact with the liquid. Such contamination not only stains common surfaces in every-day life but, when proteins or bacteria are present in the liquid, imposes severe threats to public health by seeding the formation of biofilms, a major source of infections in hospitals [20] , [37] , [38] . Moreover, the adsorption of matter from liquids onto the surface can change the surface chemistry and lead to a degradation of tailored surface properties, for example, its superhydrophobicity [15] , [39] . If direct contact of the liquid to the substrate is avoided, adsorption of contaminants to its surface can be prevented. We demonstrate that lubricated inverse monolayer substrates extremely reduce the adsorption of a variety of liquid-borne contaminants, caused by the absence of contact points between the contaminated liquid and the solid surface due to the presence of the lubricant layer, which provides a slippery, defect-free liquid/liquid interface. 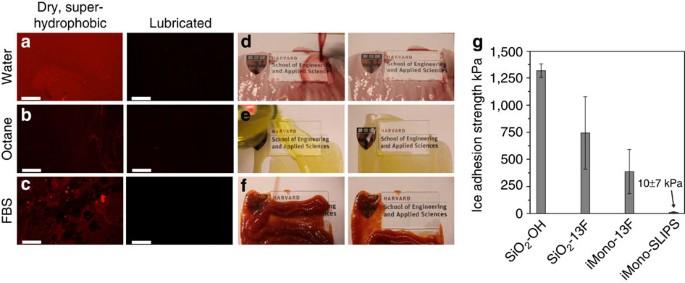Figure 3: Prevention of adhesion of different liquid-borne contaminants and reduction of ice adhesion. (a–c) Fluorescent images of the surfaces after contact with Rhodamine B in water (a), a commercially available dye (DFSB-K175) in octane (b) and Sypro Ruby-stained surfaces after incubation with undiluted fetal bovine serum (FBS) (c). Left and right images show the dry, superhydrophobic samples and the lubricated, super-repellent substrates, respectively. All surfaces were patterned with 415 nm colloid templates. All scale bars are 200 μm. (d–f) Self-cleaning and anti-staining performance of super-repellent transparent windows. The pictures are still frames fromSupplementary Movie 4demonstrating the effective repellency of wine (d), olive oil (e) and ketchup (f) from transparent SLIPS surfaces. Note significant staining of the surrounding, non-slippery surfaces. (g) Comparison of ice adhesion strength for a plain, hydrophilic glass slide (SiO2-OH); fluorosilanized, flat glass (SiO2-13F); dry, fluorosilanized inverse monolayer coating on glass (iMono-13F) and the lubricated, fluorosilanized inverse monolayer (iMono-SLIPS). All samples were made from 400-nm colloids and averaged over 10 individual measurements. The error bars represent the standard deviation of 10 individual measurements. Figure 3a–c presents fluorescence microscopy images of fluorinated, superhydrophobic inverse-monolayer surfaces without (upper row) and with (lower row) lubricant after exposure to dyed water (a), octane (b) and undiluted fetal bovine serum (c). All superhydrophobic samples failed to prevent adhesion: even though they feature high water repellency, a direct contact between the liquid and the solid cannot be avoided, leading to a rapid adsorption of liquid-borne contaminants to the hydrophobic surface [14] . In comparison, the lubricated, SLIPS samples showed negligible contamination. We envision the resistance of this transparent surface coating to protein adhesion will have a strong impact on the design of non-fouling optical windows in biomedical devices, but focus here on simple consumer applications by demonstrating the effective repellency and complete absence of staining of SLIPS-modified glass slides after spilling of red wine, olive oil and ketchup ( Fig. 3d–f , Supplementary Movie 4 ). Figure 3: Prevention of adhesion of different liquid-borne contaminants and reduction of ice adhesion. ( a – c ) Fluorescent images of the surfaces after contact with Rhodamine B in water ( a ), a commercially available dye (DFSB-K175) in octane ( b ) and Sypro Ruby-stained surfaces after incubation with undiluted fetal bovine serum (FBS) ( c ). Left and right images show the dry, superhydrophobic samples and the lubricated, super-repellent substrates, respectively. All surfaces were patterned with 415 nm colloid templates. All scale bars are 200 μm. ( d – f ) Self-cleaning and anti-staining performance of super-repellent transparent windows. The pictures are still frames from Supplementary Movie 4 demonstrating the effective repellency of wine ( d ), olive oil ( e ) and ketchup ( f ) from transparent SLIPS surfaces. Note significant staining of the surrounding, non-slippery surfaces. ( g ) Comparison of ice adhesion strength for a plain, hydrophilic glass slide (SiO 2 -OH); fluorosilanized, flat glass (SiO 2 -13F); dry, fluorosilanized inverse monolayer coating on glass (iMono-13F) and the lubricated, fluorosilanized inverse monolayer (iMono-SLIPS). All samples were made from 400-nm colloids and averaged over 10 individual measurements. The error bars represent the standard deviation of 10 individual measurements. Full size image The strong adhesion of ice to most common surfaces, causing safety and economic issues in any technology subjected to sub-zero environments, is another example where the direct contact of the material with the substrate is the principal cause for its detrimental effects. We recently demonstrated that SLIPS coatings based on highly textured polypyrrole drastically lower strength of ice adhesion to aluminium substrates [21] . Of further importance is the ability to impart transparency to such ice-repellent coatings. Figure 3g compares the adhesion strength of ice (measured at −40 °C using a custom ice adhesion setup adapted from literature) [21] , [40] for different glass substrates. The strong adhesion of ice to hydrophilic glass (1318±63 kPa) decreases with fluorination of the surface but is still substantial (743±334 kPa). The presence of a superhydrophobic, fluorinated inverse monolayer structure further decreases the ice adhesion strength (387±204 kPa). The addition of a lubricant to form a SLIPS coating drastically reduces the adhesion of ice by more than one order of magnitude compared to the superhydrophobic substrate (by decoupling the ice formation from the solid substrate). The measured ice adhesion strength on the transparent SLIPS coating (10±7 kPa) is in excellent agreement with our previous results on SLIPS coatings on aluminium [21] , suggesting that the surface properties are governed by the lubricant layer and not the solid substrate itself. Patterned wetting properties The uniformity and low height of the structures enables the application of conventional photolithographic processes to prepare locally confined patterned SLIPS regions ( Fig. 4a ). The process is based on the creation of surface functionality patterns. The lubricant is only locked-in firmly in areas with matching surface chemistry, while it will be replaced by a second liquid in areas with different surface chemistry. However, due to its low surface energy, addition of the lubricant leads to a homogeneous lubricant film covering the entire coating. Upon addition of a second liquid, a metastable state can be created in which the lubricant layer is not immediately disrupted by the applied liquid ( Fig. 4a ). Eventually, the energetically most favourable state is reached as the liquid displaces the lubricant layer in non-functionalized surface regions. Stable SLIPS surface regions defined by the fluorinated surface chemistry remain wetted solely by the lubricant. 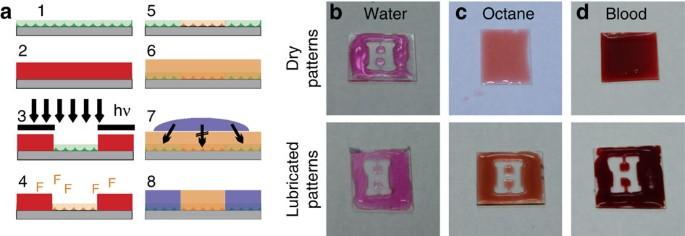Figure 4: Patterning of transparent repellent surfaces. (a) Photolithographic patterning of nanostructured samples to create SLIPS patterns based on matching surface functionalities: An inverse monolayer substrate (1) is coated with photoresist (2), irradiated and developed to create the desired surface pattern (3). Vapor-phase fluoro silanization is applied to create fluorinated surface functionalities at the exposed surface regions (4); the protected surface regions remain unfunctionalized after removal of the photoresist (5). Due to its low surface energy, the lubricant first creates a homogeneous liquid film on the surface (6). Addition of a second liquid (7) that has a higher affinity to the unfunctionalized surface areas than the lubricant leads to localized replacement of the lubricant at the unfunctionalized surface areas (8). (b–d) Patterning of various liquids based on surface chemistry contrasts. The upper row shows the addition of liquids to the dry, patterned substrates (after step 5 of the scheme shown in (a)). The lower row shows the addition of liquids to the pre-lubricated substrates (following the full process shown in (a)). (b) Rhodamine B-dyed water: the pattern is revealed both in a dry state and on the lubricated sample; (c) DFSB-K175-dyed octane and (d) sheep blood: the liquids wet and contaminate the entire surface in a dry state, while successful patterning occurs using the repellent properties of SLIPS surface areas. Figure 4: Patterning of transparent repellent surfaces. ( a ) Photolithographic patterning of nanostructured samples to create SLIPS patterns based on matching surface functionalities: An inverse monolayer substrate (1) is coated with photoresist (2), irradiated and developed to create the desired surface pattern (3). Vapor-phase fluoro silanization is applied to create fluorinated surface functionalities at the exposed surface regions (4); the protected surface regions remain unfunctionalized after removal of the photoresist (5). Due to its low surface energy, the lubricant first creates a homogeneous liquid film on the surface (6). Addition of a second liquid (7) that has a higher affinity to the unfunctionalized surface areas than the lubricant leads to localized replacement of the lubricant at the unfunctionalized surface areas (8). ( b – d ) Patterning of various liquids based on surface chemistry contrasts. The upper row shows the addition of liquids to the dry, patterned substrates (after step 5 of the scheme shown in ( a )). The lower row shows the addition of liquids to the pre-lubricated substrates (following the full process shown in ( a )). ( b ) Rhodamine B-dyed water: the pattern is revealed both in a dry state and on the lubricated sample; ( c ) DFSB-K175-dyed octane and ( d ) sheep blood: the liquids wet and contaminate the entire surface in a dry state, while successful patterning occurs using the repellent properties of SLIPS surface areas. Full size image The superior performance of the SLIPS-based approach to create patterns of liquids on solid substrates is revealed in Fig. 4b–d and in Supplementary Movies 5 and 6 . The figure shows the successful confinement of several test liquids to designated surface regions based on matching surface chemistry. Owing to its high surface tension, water can be confined to hydrophilic surface regions on a dry, patterned substrate as well as with the SLIPS-based approach ( Fig. 4b ). An advantage of the latter is the prevention of adhesion of contaminants from the water phase that cannot be excluded for the dry patterning approach (compare to Fig. 3 ). Octane, as a low-surface-tension test liquid ( Fig. 4c ), and sheep blood, as an example of a complex fluid ( Fig. 4d ), fail to be confined on the dry, patterned substrate: both liquids wet the entire surface, whereas a clear pattern can be resolved in the SLIPS-based approach. The creation of patterns of such fluids is extremely challenging with state-of-the-art coatings. Assessment of thermodynamic stability and defect tolerance Compared to existing approaches to creating nanoscale surface patterns [19] , [21] , [24] , the design of SLIPS coatings using a simple, bottom-up colloidal self-assembly process produces surface structures with finely controlled feature sizes, high regularity and uniformity. This allows us to analyze and compare the stability of the transparent SLIPS coatings with theoretical predictions based on thermodynamic considerations, and thus advance the fundamental understanding of the surface properties and function. We start by calculating the minimum surface roughness R— defined as the ratio of the surface area of the porous substrate to that of a flat surface — required to support a stable SLIPS condition based on the surface energy balance concept [19] , [23] . The stability of a system with a droplet of liquid A (contact angle θ A , surface tension γ A ) sitting on top of a film of lubricant B ( θ B , γ B ; interfacial tension of the two liquids γ AB ) is predicted by [19] : For octane as droplet and DuPont Krytox 100 as lubricant, we yield R >1.51±0.1 as the threshold value to support stable SLIPS ( Supplementary Note 1 ). A geometric analysis of the inverse monolayer structure estimates the roughness factor to be 1.91 ( Supplementary Note 1 ). Hence, a uniform inverse colloidal monolayer is indeed capable of supporting a thermodynamically stable configuration. Additionally, it is worth noting that SLIPS stability, as predicted by the equation, is not a function of the actual structure size, thus providing the thermodynamic foundation for the design of completely transparent coatings based on increasingly small feature sizes. In applications, it is critical to understand the defect tolerance and the associated thermodynamic penalties of imperfect or damaged SLIPS coatings. The inverse monolayer substrates provide a perfect system to assess these parameters. By varying the amount of tetraethylorthosilicate (TEOS) used for the inverse monolayer preparation, it is possible to tune the surface coverage of the nanostructures from an intact inverse monolayer to highly damaged surfaces featuring only small monolayer patches ( Fig. 5a , Supplementary Fig. S5 ). The length scale of the defects on the substrates is on the order of few micrometres ( Supplementary Fig. S6 ) and, hence, small compared to the dimension of a macroscopic liquid droplet. Thus, the droplet experiences a total roughness that is averaged from intact inverse monolayer and monolayer-free areas. We systematically adjusted the total roughness of surfaces from 1.0 (flat, unstructured glass surface) to 1.91 (intact structure) and, after fluorosilanization and addition of a lubricant, investigated their performance in repelling octane ( Fig. 5d ). All structured samples show effective octane repellency, as indicated by very small sliding angles (<5°). Comparing the roughness values in the experiment with the calculated minimum surface roughness, we conclude that the more damaged samples support a metastable SLIPS coating that, even though not in its thermodynamically stable state, sustain their repellent character, at least over the time frame of the experiment and in the absence of any external stresses. Placement of an octane droplet onto the substrates over a longer time (>15 min) revealed pinning for the most damaged sample ( R =1.14), while all other substrates remained repellent, corroborating metastability of the coating in short-term applications. We further note that while the thermodynamic calculations are derived from the four-phase substrate/lubricant/liquid/air system, a more fundamental requirement for SLIPS is the ability of the lubricant to wet the surface homogeneously (that is, apparent contact angle θ * =0°). Using Wenzel’s relation (cos θ * =R cos θ ) [41] , we calculate the minimum roughness needed for complete wetting to be 1.11 ( θ Krytox =26.1°). Thus, we attribute the unexpected repellent behavior of highly damaged samples to their ability to support homogeneous wetting of the lubricant, the replacement of which by the probe liquid is slow compared to the experimental time frame. By virtue of the same argument, the flat sample fails to support high repellency because it is not completely wetted by the lubricant and thus exposes dry, de-wetted areas to which the octane droplet adheres ( Fig. 5d , insets). 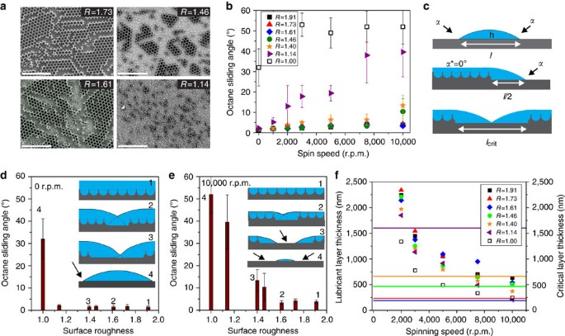Figure 5: Assessment of the stability of transparent SLIPS coatings. (a–f) Effect of damage in the porous layer on liquid repellency: (a) SEM images of substrates with varying inverse monolayer surface coverage. All scale bars are 10 μm. (b) Octane sliding angles measured on samples with varying amount of damage subjected to spin-coating to thin out the lubricant layer. All values were averaged over 10 individual measurements. The error bars represent the standard deviation of 10 individual measurements. (c) Schematic illustration of the effect of defect structures on the lubricant meniscus. On a flat substrate, a finite contact angleαgives rise to partial wetting with a contact lengthl(top). The presence of surface roughness leads to complete spreading of the lubricant (α*=0°). At the edge of the roughness feature, the droplet will extend onto the unstructured region byl/2(middle). A defect between two roughened areas can therefore sustain a homogeneous lubricant film up to a critical length oflcrit(bottom). (d) Performance in octane repellency before spin-coating. All structured samples, even with low area coverage of inverse monolayer structures (that is, lower surface roughness), show effective octane repellency, while a smooth surface shows significant pinning. The inset shows the wetting situation for the different structures schematically. Pinning points are indicated by an arrow. (e) Performance in octane repellency after spin-coating at 10,000 r.p.m. Only samples with roughness values of >1.61 retain their repellent character. The decrease in lubricant layer thickness leads to exposure of the substrate for larger defect structures (insets). All values were averaged over 10 individual measurements. The error bars represent the standard deviation of 10 individual measurements. (f) Comparison of the critical lubricant layer thickness calculated for the different defect structures (details inSupplementary Note 2) with the actual lubricant layer thickness during spin-coating. Stable repellency is expected as long as the measured layer thicknesses (data points) remain above the critical theoretical threshold (lines). Figure 5: Assessment of the stability of transparent SLIPS coatings. ( a – f ) Effect of damage in the porous layer on liquid repellency: ( a ) SEM images of substrates with varying inverse monolayer surface coverage. All scale bars are 10 μm. ( b ) Octane sliding angles measured on samples with varying amount of damage subjected to spin-coating to thin out the lubricant layer. All values were averaged over 10 individual measurements. The error bars represent the standard deviation of 10 individual measurements. ( c ) Schematic illustration of the effect of defect structures on the lubricant meniscus. On a flat substrate, a finite contact angle α gives rise to partial wetting with a contact length l (top). The presence of surface roughness leads to complete spreading of the lubricant ( α *=0°). At the edge of the roughness feature, the droplet will extend onto the unstructured region by l/2 (middle). A defect between two roughened areas can therefore sustain a homogeneous lubricant film up to a critical length of l crit (bottom). ( d ) Performance in octane repellency before spin-coating. All structured samples, even with low area coverage of inverse monolayer structures (that is, lower surface roughness), show effective octane repellency, while a smooth surface shows significant pinning. The inset shows the wetting situation for the different structures schematically. Pinning points are indicated by an arrow. ( e ) Performance in octane repellency after spin-coating at 10,000 r.p.m. Only samples with roughness values of >1.61 retain their repellent character. The decrease in lubricant layer thickness leads to exposure of the substrate for larger defect structures (insets). All values were averaged over 10 individual measurements. The error bars represent the standard deviation of 10 individual measurements. ( f ) Comparison of the critical lubricant layer thickness calculated for the different defect structures (details in Supplementary Note 2 ) with the actual lubricant layer thickness during spin-coating. Stable repellency is expected as long as the measured layer thicknesses (data points) remain above the critical theoretical threshold (lines). Full size image The substrates were also subjected to high shear forces induced by spin-coating at increasing rotational speeds ( Fig. 5b ). Figure 5e shows the resulting octane sliding angles after the final step of spin-coating at 10,000 r.p.m. Remarkably, substrates with a roughness of >1.61 did not lose their repellency and showed low sliding angles <5°, implying the presence of an intact lubricant layer completely covering the porous solid ( Fig. 5e , insets 1–2). All other samples showed increased sliding angles, indicating partial loss of the lubricant layer at the damaged parts of the substrate and subsequent pinning of octane at the exposed solid surface ( Fig. 5e , insets 3, 4). To demonstrate the superior performance of the presented coating, an open-cell epoxy micropillar sample [19] was subjected to the same spin-coating protocol and failed to retain its repellency after 2,000 r.p.m. ( Supplementary Fig. S7 ). We established a simple model to predict the onset of lubricant de-wetting caused by a defect between regular surface structures ( Fig. 5c ). The model correlates the critical defect length l crit (the maximum defect length that supports complete lubricant coverage) with the thickness h and the contact angle of the lubricant on the solid substrate ( Supplementary Note 2 , Supplementary Figures S8–S11 ): Figure 5f compares the experimentally measured lubricant layer thicknesses after the individual spin-coating steps (data points) to the calculated critical lubricant thicknesses (solid lines). Once the measured thickness drops below the theoretically calculated value, de-wetting and hence failure to repel octane is expected. A comparison between the predicted and measured repellency failures yielded an excellent agreement ( Table 1 ). Thus, our simple model accurately explains and predicts stable repellency or failure for any given damaged sample at all different spinning speeds. Table 1 Comparison of measured and predicted repellency failure upon spin-coating at different spinning speeds. Full size table The experiments reveal a remarkable affinity of the lubricant layer to the porous surface. Samples with a substantial amount of damage (up to 33% of the complete surface) continuously support repellency even at the maximum rotational speeds available in our setup. This has important consequences for creating robust coatings for industrial and consumer applications. We further note that our thermodynamically stable coatings maintain their repellency over an extended period of time, which we confirmed by the long-term stability of octane repellency on vertically stored substrates, mimicking an actual window ( Fig. 6a ). Even after >9 months of vertical storage without replenishment of lubricant, all samples continue to show octane sliding angles well below 10°. Moreover, the closed-cell architecture of the inverse monolayer paired with the efficient, covalent binding of the silica sol–gel on glass adds superior mechanical stability to the nanoscale coating. 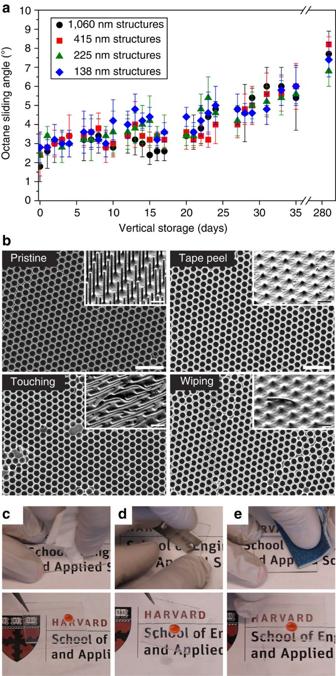Figure 6: Long-term stability and mechanical robustness of the transparent coating. (a) Long-term storage of glass slides covered with lubricated nanostructures in a vertical orientation. Even after extended storage time exceeding 9 months without lubricant replenishment, all samples showed high octane repellency with low sliding angles. All values were averaged over 10 individual measurements. The error bars represent the standard deviation of 10 individual measurements. (b) Mechanical stability of the closed-cell, inverse monolayers shown by SEM images of surface structures after subjection to different mechanical treatments. The inverse monolayer coating withstands touching, wiping and tape peel tests, while open-cell reference samples (epoxy micropillars; shown for comparison as insets) are completely damaged by all treatments. All scale bars are 5 μm. (c–e) Mechanical robustness and self-healing properties of transparent, super-repellent glass slides that show efficient repellency of a dyed octane droplet maintained after mechanical wiping (c), scratching with a razor blade (d) and sandpaper (e) (still frames taken fromSupplementary Movie 7). Figure 6b demonstrates the complete structural integrity of inverse monolayer samples after being subjected to a variety of mechanical treatments including touching, wiping and tape peel tests. An open-cell reference sample consisting of epoxy micropillars was completely destroyed by any of the treatments ( Fig. 6b , insets). The combination of high mechanical stability of the structures ( Fig. 6b ), damage tolerance of the lubricant-infused coating ( Fig. 5b ) and the unique self-healing properties arising from the liquid nature of the lubricant [19] suggests that the surfaces can tolerate various mechanical treatments likely to occur in daily-life applications. In Fig. 6c–e , we present still frames taken from Supplementary Movie 7 demonstrating the retention of high repellency after mechanical damage induced by cleaning with a tissue (c), scratching with a razor blade (d) and treatment with sandpaper (e). Figure 6: Long-term stability and mechanical robustness of the transparent coating. ( a ) Long-term storage of glass slides covered with lubricated nanostructures in a vertical orientation. Even after extended storage time exceeding 9 months without lubricant replenishment, all samples showed high octane repellency with low sliding angles. All values were averaged over 10 individual measurements. The error bars represent the standard deviation of 10 individual measurements. ( b ) Mechanical stability of the closed-cell, inverse monolayers shown by SEM images of surface structures after subjection to different mechanical treatments. The inverse monolayer coating withstands touching, wiping and tape peel tests, while open-cell reference samples (epoxy micropillars; shown for comparison as insets) are completely damaged by all treatments. All scale bars are 5 μm. ( c – e ) Mechanical robustness and self-healing properties of transparent, super-repellent glass slides that show efficient repellency of a dyed octane droplet maintained after mechanical wiping ( c ), scratching with a razor blade ( d ) and sandpaper ( e ) (still frames taken from Supplementary Movie 7 ). Full size image We conclude by briefly discussing the characteristic properties of the lubricant-infused inverse monolayer-based coating. The surfaces combine all the attractive properties of previously reported SLIPS coatings, including highly effective liquid repellency toward a variety of liquids, prevention of contamination and a strong decrease of ice adhesion strength. The process can be scaled and allows coating of curved substrates. The size of the pores can be tuned over a wide range, and can be designed to be small enough to not interfere with light of visible wavelengths and even to enhance the transmission of light, leading to omniphobic, optically clear coatings required in many applications where transparency of the surface is critical. The coating exhibits remarkably robust surface structures, resulting from the interconnected pore geometry of the inverse monolayer paired with the stable, covalent adhesion of the silica scaffold to oxide surfaces. Its repellent character is retained after extended periods of time and repellency prevails after the application of strong shear forces and mechanical damage. The methodology is compatible with conventional patterning processes, which can be used to create locally confined SLIPS patterns on a substrate, allowing confinement of low-surface-tension liquids and complex fluids to designated surface areas. In addition to the demonstrated performance characteristics of these surfaces, their high uniformity and order coupled with the ability to regulate the defect distribution allow for precise control of the surface roughness and comparison of the stability of the SLIPS coating with theoretical predictions, leading to a deeper insight into the mechanisms of wetting occurring on SLIPS surfaces. We show that the lubricant-infused inverse monolayers are thermodynamically stable for intact structures while heavily damaged structures can support a metastable repellency state. Furthermore, we develop a simple geometric model that can be applied to predict the stability or failure of the coating as a function of the lubricant layer thickness and the size of defects in the samples. All these characteristics add to a versatile surface coating with an unprecedented combination of properties. A wide variety of applications of the presented technology can be envisioned, including omniphobic, self-cleaning and self-healing windows or solar panels, face shields, glasses, goggles or lenses and non-fouling windows or surface patterns in biomedical diagnostic assays or devices. Formation of colloidal monolayers on glass Colloidal monolayers were crystallized on the air–water interface of a crystallization dish following a protocol from literature [34] . Briefly, a colloidal dispersion in 1:1 water/ethanol (solid content ~2.5%) was spread onto the interface via a glass slide until the surface was completely covered. The substrate was then inserted into the subphase and the monolayer was deposited manually by fishing out the slide. After drying, a closed-packed monolayer uniformly covered the substrate. All colloids were prepared by surfactant-free emulsion polymerization of styrene with acrylic acid as comonomer. Formation of the inverse monolayer A solution of tetraethylorthosilicate (TEOS), HCl (0.1 mol l −1 ) and ethanol with weight ratios of 1:1:1.5 was prepared and stirred for 1 h. Then, it was diluted with ethanol (for dilution ratios, see Supplementary Table S1 ) and spin-coated onto the monolayer-covered substrate (3,000 r.p.m., 30 s, acceleration 500). The colloids were removed by combustion at 500 °C (ramped from RT to 500 °C for 5 h, 2 h at 500 °C). To prepare damaged surfaces, the TEOS concentration was systematically decreased as specified in Supplementary Table S2 . Fluorosilanization Fluorosilanization was carried out by vapor-phase deposition of (1H,1H,2H,2H-tridecafluorooctyl)-trichlorosilane (or Decyltrichlorosilane) for 24 h at reduced pressure and room temperature. Prior to silanization, the substrates were cleaned in acid piranha (3:1 sulphuric acid:hydrogen peroxide; warning: reacts very violently with organic materials) and plasma-treated with oxygen plasma for 10 min. Lubrication 10 μl cm −2 Krytox 100 (or similar amounts of water or olive oil) was added to the substrate and uniform coverage was achieved by tilting. Excess lubricant can be removed by vertical placement of the substrates. For the long-term experiment, the more viscous Krytox 103 was used to minimize the evaporation of the lubricant. Patterning A conventional photoresist (S1818, positive tone resist) was spin-coated (4,000 r.p.m., 60 s) on the unsilanized inverse monolayer substrate. Illumination with UV light was performed by following the recipe of the photoresist manufacturer (Shipley Company, Marlborough, MA) with an irradiation dose of 200 mJ cm −2 followed by development of the structures (Developer MF319, 60 s). The substrate, consisting of areas covered by photoresist and free areas was plasma-treated for 5 min and then fluorosilanized similar to non-patterned substrates. After silanization, the resist was washed off the substrate (Remover PG 1165). The application of a lubricant then produced patterned SLIPS surfaces, as the conditions for a stable SLIPS state is only fulfilled in the fluorosilane-functionalized surface regions. Contact-angle measurements The contact-angle measurements were performed with a contact-angle measurement system (KSV CAM 101) at room temperature with ~20% relative humidity. The droplet volume for the measurements was 5 μl (unless otherwise specified) and the macroscopic droplet profile was captured through a camera. The droplet profile was fitted into a spherical cap profile by a computer programme provided by the manufacturer of the system. Contact-angle hysteresis was measured by increasing and decreasing the droplet volume while taking screenshots and extracting the advancing and receding contact angles. Sliding angles were measured on a customized tilting stage with a droplet volume of 20 μl. All contact angle values specified in the text were averaged over at least 10 individual measurements. Mechanical stability tests The mechanical stability was assessed by (i) pressing a finger onto the surface structures, (ii) vigorously wiping it with an ethanol-soaked tissue, (iii) scratching with the razor-blade or sandpaper, and (iv) applying Scotch Tape to the coating followed by peeling off the tape. After the treatments, all surface structures were imaged by SEM. How to cite this article: Vogel, N. et al . Transparency and damage tolerance of patternable omniphobic lubricated surfaces based on inverse colloidal monolayers. Nat. Commun. 4:2176 doi: 10.1038/ncomms3176 (2013).